Direct writing of electronic devices on graphene oxide by catalytic scanning probe lithography Reduction of graphene oxide at the nanoscale is an attractive approach to graphene-based electronics. Here we use a platinum-coated atomic force microscope tip to locally catalyse the reduction of insulating graphene oxide in the presence of hydrogen. Nanoribbons with widths ranging from 20 to 80 nm and conductivities of >10 4 S m −1 are successfully generated, and a field effect transistor is produced. The method involves mild operating conditions, and uses arbitrary substrates, atmospheric pressure and low temperatures (≤115 °C). Graphene, owing to its exceptionally high carrier mobility, has been envisioned as one of the best candidates for future electronics [1] , [2] , [3] , [4] , [5] , [6] , [7] . The possibility of direct writing on graphene to construct electronic circuits by scanning probe lithography (SPL) is particularly exciting and has been extensively examined by different approaches [8] , [9] , [10] , [11] with the focus of creating well-defined insulated separators on highly conductive graphene. In this context, a chemically more realistic approach is to create conducting nanoribbons on insulated graphene oxides (GO) through the reduction reaction. GO has been used as the seed for cost-effective mass production of graphene in recent years [12] , [13] , [14] , [15] . The conductivity of a fully oxidized GO is extremely small, but it can be significantly increased by chemical reduction [13] , [16] . Such a contrast offers the opportunity to utilize direct writing of electronic circuits on GO if an efficient local chemical reduction process can be obtained. Recently, it is reported that the direct writing with nanoscopic resolution can be achieved through local thermal reduction of GO with a heated atomic force microscope (AFM) tip [17] . However, the maximal contrast can only be reached at a temperature around 1000 °C [17] , which might be too high for practical applications. It is highly desirable to find a local reduction scheme [18] that works at much more mild conditions. For this purpose, a highly efficient catalysed reaction should be introduced through the use of the catalytic SPL (cSPL) technique [19] , [20] , [21] , [22] . Here we demonstrate the feasibility of the cSPL technique for the direct writing of electronic circuits on GO. It is accomplished by using a Pt-coated AFM tip to locally catalyse the reduction reaction of GO with hydrogen. This technique allows the efficient generation of highly conductive crossed nanoribbons, as well as prototype ambipolar field effect transistors (FETs) with arbitrary substrates, under atmospheric pressure and at low temperatures (≤115 °C). Local reduction of GO via the cSPL under mild conditions We have found that by using a Pt-coated AFM tip with the assistance of hydrogen gases, the reaction barrier for GO reduction can be significantly reduced and high conductivity contrast with nanoscopic resolution can be obtained at a temperature ≤115 °C under atmospheric pressure. Our experimental setup is schematically shown in Fig. 1a , in which the monolayer GO sheet was pre-dispersed on an insulating substrate with one side connected to the gold pad. After the AFM tip is scanned on the sample at 100 °C in the presence of hydrogen gases with a load force of 10 nN and a scanning speed of 1 nm s −1 , a shallow groove, which is 80 nm wide and 2 μm long, can be observed from the topographical images shown in Fig. 1b and c . This groove appears to be a very bright nanoribbon in the scanned current image, which was measured under a bias voltage of 2 V between the gold electrode and the conducting tip scanned over the area in Fig. 1d . It clearly indicates that the nanoribbon is conductive (with the current overranging 100 nA as limited by our SPM equipment), whereas the other area remains insulated. As the substrate is insulating, this huge contrast in the conductance firmly demonstrates that the nanoribbon is reduced GO (rGO). The current–voltage ( I–V ) characteristics measured at the different positions on the nanoribbon are given in Fig. 1e . The resistance ( R ) is found to be linearly dependent on the length ( L ) of the nanoribbon as defined by the distance from the measured point to the gold electrode, obeying the simple Ohm’s law. This allows us to calculate the resistivity and the conductivity of the nanoribbon. The conductivity of the nanoribbon is estimated to be about 10 3 S m −1 , which is within the same order of magnitude as that for chemically rGO [23] , [24] and is much larger than that for GO. 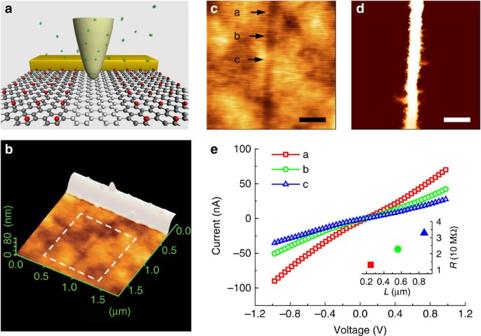Figure 1: The local reduction scheme of GOviathe cSPL and its implementation. (a) The experimental setup of the cSPL. A rGO nanoribbon is written at 100 °C perpendicularly to the gold electrode laid on one end of the GO sheet. (b) Three-dimensional topographical AFM image of the GO sheet after the writing. (c) The topographical image of the marked area in (b). (d) Current image at a sample bias of 2 V with a colour scale (black to white) of 100 nA. (e) TheI–Vcurves measured at the three spots marked in (c), the inset shows the relationship between the length and the resistance of the nanoribbon. The scale bars in (c,d) are both 200 nm. [16] Figure 1: The local reduction scheme of GO via the cSPL and its implementation. ( a ) The experimental setup of the cSPL. A rGO nanoribbon is written at 100 °C perpendicularly to the gold electrode laid on one end of the GO sheet. ( b ) Three-dimensional topographical AFM image of the GO sheet after the writing. ( c ) The topographical image of the marked area in ( b ). ( d ) Current image at a sample bias of 2 V with a colour scale (black to white) of 100 nA. ( e ) The I – V curves measured at the three spots marked in ( c ), the inset shows the relationship between the length and the resistance of the nanoribbon. The scale bars in ( c , d ) are both 200 nm. Full size image We have also performed two control experiments to examine the roles of the Pt-coated tip and the hydrogen gases. In one of them, the AFM tip was replaced with a fresh silicon tip or a gold-coated tip, whereas in the other the sample was placed in a low-vacuum environment without hydrogen atmosphere. All other conditions were kept the same. As expected, the groove pattern of nanoribbon cannot be observed in both topographical and friction images after scanning ( Supplementary Figs S1 and S2 ). This result shows that both Pt-coated tip and hydrogen gases are indispensably involved in the reduction of GO. This view has been further verified by X-ray photoelectron spectroscopy, and the results are given in Supplementary Fig. S3 . The effects of the load force and the scanning speed of the tip as well as the temperature of the substrate on the reduction reaction are also shown in Supplementary Figs S4 and S5 . 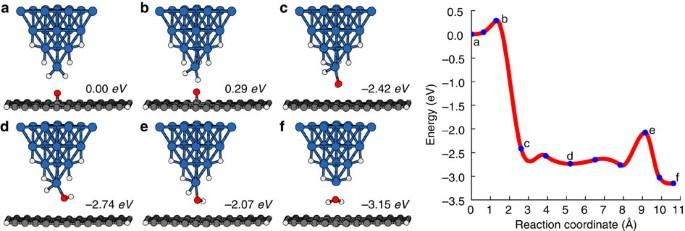Figure 2: Computational models and the energy profile for the catalysed reduction reaction process. The corresponding structures for the reduction process of the GO (described by monolayer graphene with an epoxy group on it) are marked by (a–f). The red line in the right profile is fitted according to the energy and force (first derivative of energy) of each image (blue dots marked bya–f). The big blue, medium red, medium grey and small white spheres represent Pt, O, C and H atoms, respectively. Density functional theory calculations Figure 2 gives the computational models and the energy profile for the catalysed reduction reaction process of an epoxy group on monolayer graphene. Considering that the hydrogen molecules can be dissociated by a Pt tip to form platinum hydride [25] , [26] , we believe that the reduction process goes in two steps according to our calculations. First, the oxygen atom gradually moves away from the GO and approaches towards the hydrided Pt tip. After overcoming an energy barrier of about 0.29 eV, the oxygen and a hydrogen atoms form a hydroxyl group, which is chemically bonded to the Pt tip. In the second step, this hydroxyl group gets close to the other hydrogen atoms. A water molecule forms and finally desorbs from the tip. Although the energy barrier of the second step is estimated to be as high as 0.67 eV, the large energy release of 2.74 eV from the first step makes it quite feasible to overcome this barrier. While moving towards the next epoxy group, the tip is hydrided again by the dissociative adsorption of hydrogen molecules and a new cycle of GO reduction begins. It is also found that the hydroxyl group is easier to be reduced than the epoxy group as its energy barrier is only about 0.10 eV for the first step. Another important factor that controls the reaction rate is the distance between the tip and the oxidation groups on the GO. A larger distance can result in the increase of the energy barrier for the first step. Figure 2: Computational models and the energy profile for the catalysed reduction reaction process. The corresponding structures for the reduction process of the GO (described by monolayer graphene with an epoxy group on it) are marked by ( a – f ). The red line in the right profile is fitted according to the energy and force (first derivative of energy) of each image (blue dots marked by a – f ). The big blue, medium red, medium grey and small white spheres represent Pt, O, C and H atoms, respectively. Full size image Direct writing highly conductive rGO nanoribbons With this technique, we are ready to write more complicated nanopatterns on GO. As a demonstration, crossed conducting rGO nanoribbons are generated and shown in Fig. 3a . A main path of an 81-nm-wide nanoribbon is first generated, which is perpendicularly connected with the gold electrode. Three parallel nanoribbons, with the widths of 61, 32, and 20 nm, respectively, are then written to cross over the main path. The corresponding current image generated at a bias of 0.5 V is well illustrated in Fig. 3b . Eight spots, as marked in Fig. 3a , have been chosen to study their electrical characteristics, and the measured I – V curves are plotted in Fig. 3c . By assuming the contact resistance between the tip and the rGO to be a constant, the resistance per length ( R/L ) of the ribbon as the function of the width ( W ) is estimated and shown in the inset of Fig. 3c . As seen, the electrical characteristics of the nanoribbons largely obey the Ohm’s law: for the three wide ribbons, the resistance per length is almost inversely proportional to the width; whereas the result for the 20-nm ribbon shows an obvious deviation. The latter could be due to the slight discontinuation of the nanoribbon, as illustrated in Fig. 3b . Furthermore, the average line profiles of the height and the current in Fig. 3d clearly indicate that this technique is capable of writing ~20-nm-wide nanopatterns. 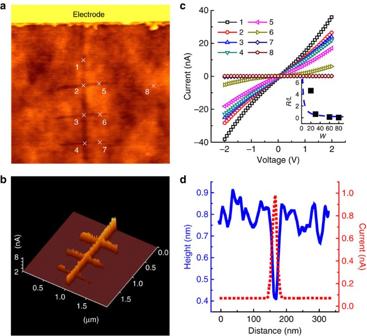Figure 3: Electrical characteristics of crossed rGO nanoribbons fabricated at 100 °C. (a) The topographical image of the crossed nanopattern. (b) The three-dimensional current image obtained at 0.5 V. The colour scale is 15 nA. (c) TheI–Vcurves measured for eight spots, of which seven spots are on the nanoribbons and one (the eighth) is placed at the unscanned region as the reference. The inset is the relationship between the estimated resistance per length (R/L, unit: × 109Ω μm−1) and the width (W, unit: nm) of the ribbon, the blue dashed line represents an ideal inversely proportional relationship. (d) The average line profiles of the height (blue solid line) and the current (red dot line) of the 20-nm-wide nanoribbon. Figure 3: Electrical characteristics of crossed rGO nanoribbons fabricated at 100 °C. ( a ) The topographical image of the crossed nanopattern. ( b ) The three-dimensional current image obtained at 0.5 V. The colour scale is 15 nA. ( c ) The I – V curves measured for eight spots, of which seven spots are on the nanoribbons and one (the eighth) is placed at the unscanned region as the reference. The inset is the relationship between the estimated resistance per length ( R/L , unit: × 10 9 Ω μm −1 ) and the width ( W , unit: nm) of the ribbon, the blue dashed line represents an ideal inversely proportional relationship. ( d ) The average line profiles of the height (blue solid line) and the current (red dot line) of the 20-nm-wide nanoribbon. Full size image The feasibility of the proposed technique can be further demonstrated by the fabrication of a nanoribbon FET (nr-FET), as schematically shown in Fig. 4a (see Methods for details). 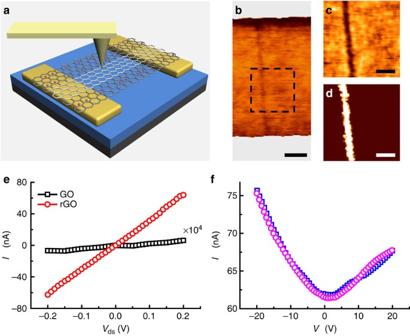Figure 4: Electrical characteristics of a 40-nm-wide rGO nanoribbon FET fabricated at 115 °C. (a) Schematic of the device. (b) The topographical image of the rGO nanoribbon bridged between two electrodes (the white areas), the scale bar is 200 nm. (c) The topographical and (d) the corresponding current images of the marked area in (b). The scale bars are 100 nm. (e) TheI–Vcurves between the two electrodes measured before (black) and after (red) the nanoribbon is written. (f) The transfer characteristic of the nanoribbon with the forward (magenta) and backward (blue) scans ofVgwhileVds=0.2 V. Figure 4b–d shows the topographical and current images of the fabricated nr-FET. The success of the writing is firmly confirmed by the huge current contrast between the nanoribbon and the surrounding. The measurement for the electrical characteristics of the FET has been carried out in vacuum at room temperature before and after the nanoribbon is produced. As shown in Fig. 4e , the source-drain current ( I ds ) is negligible in the GO FET, but it increases by five orders of magnitude after the rGO nanoribbon is written. Figure 4f shows the transfer characteristic of the nr-FET when the gate voltage ( V g ) varies from 20 to −20 V with a source-drain voltage ( V ds ) of 0.2 V. One can see that the obtained curve exhibits an obvious ambipolar behaviour. The hole mobility, slightly larger than that of the electron, is estimated to be about 21 cm 2 V −1 S −1 . Furthermore, the curve shows small hysteresis and the minimal conductance is right located around zero gate voltage. Both features indicate that the reduced graphene nanostructure has not been doped by the catalytic reduction involved. Figure 4: Electrical characteristics of a 40-nm-wide rGO nanoribbon FET fabricated at 115 °C. ( a ) Schematic of the device. ( b ) The topographical image of the rGO nanoribbon bridged between two electrodes (the white areas), the scale bar is 200 nm. ( c ) The topographical and ( d ) the corresponding current images of the marked area in ( b ). The scale bars are 100 nm. ( e ) The I – V curves between the two electrodes measured before (black) and after (red) the nanoribbon is written. ( f ) The transfer characteristic of the nanoribbon with the forward (magenta) and backward (blue) scans of V g while V ds =0.2 V. Full size image The temperature has a key role in controlling a chemical reaction. In general, a higher temperature is better even under the catalytic condition. We have carefully examined the effect of the temperature on the conductivity and mobility of the written rGO nanoribbons. It is noted that in our experimental setup, we could only be able to heat the entire sample. In this case, the window of the working temperature should be quite small as with too high temperature, the oxidation groups at the unwritten area will also be partially reduced and the current contrast will significantly decrease. The best working temperature for our experiments is 115 °C, at which the conductivity can be enhanced by more than ten times in comparison with that obtained at 100 °C ( Supplementary Fig. S6 ). A collection of the results for rGO nanoribbons written at different temperatures is given in Supplementary Figs S6 and S7 . It might be worth mentioning that our best conductivity is about 30 times of that reported in Wei et al. [17] ( Supplementary Fig. S6 ). Moreover, for our samples, the conductivity contrast is at least six orders of magnitude, as demonstrated in Supplementary Fig. S6 ; whereas only three to four orders of magnitude were obtained in the previous study [17] . The concept of using localized catalytic reaction to utilize the direct writing of electronic devices at the nanoscale on GO has been fully verified by all those convincing experimental results. This technique has a great potential to be further improved. One way to do it is to find better catalysts that can accelerate the reaction under the proper working temperature. Obviously, the ultimate solution is to combine the best of two worlds: the localized catalytic reaction proposed here and the local heating approach utilized in Wei et al. [17] Unfortunately at the moment we do not have the access to the necessary resources to manufacture such tips. To conclude, a new catalytic technique for the direct writing of electronic circuits on GO under mild experimental conditions has been demonstrated by AFM with a Pt-coated tip in a hydrogen atmosphere. The constructed nanoribbons and FET are of high quality with good functionalities. This mild, clean and straightforward technique is an important step towards the realization of grapheme-based nanoelectronics and sensing technologies. cSPL experiments The cSPL [18] , [19] , [20] , [21] , [22] adopted in our study was carried out on monolayer GO sheets, it takes several steps to prepare them. The GO powder was first prepared by the oxidative treatment of graphite (high purity of 99.9999%, 200 mesh, Alfa-Aesar) with the modified Hummers method [14] . This GO powder was redissolved in milli-Q water and then centrifuged to remove the residual large particles. The concentration of the GO solution was controlled to be 0.01%. After that, a 5 μl of the solution was dropped onto the substrates (SiO 2 or sapphire). To keep the GO sheets lay on the substrates without crinkles, the droplet was slowly evaporated, thus resulting in large-area, smooth monolayer GO sheets free of nanoscale wrinkling. Before writing with cSPL or any measurement, the samples were heated in nitrogen atmosphere to 100–115 °C for 15 min to remove the residual solvent and water. The cSPL writing was performed on a SPA400 instrument with a SPI-3800 controller (Seiko Instrument Industry Co.). A commercial Pt-coated tip with force constant of 0.2 N m −1 was used. The chamber was filled with 99.999% hydrogen at a pressure of 0.1 MPa. The hydrogen molecules were injected through a mass flow controller with the speed of 0.5 standard liter per minute. The temperature of the substrates was controlled by a heat stage and the accuracy is within ±1 °C. The Pt-coated AFM tip was set to scan on the GO surface in the vector scan mode with controlled speeds and forces. To fabricate the prototype nr-FET, a pair of Au/Ti (20/10 nm or 10/10 nm) source and drain electrodes (channel length ~1000, nm) have been fabricated by e-beam lithography on a 300-nm-thick SiO 2 /Si (heavily doped, which serves as the back gate) substrate. A monolayer GO sheet was then smoothly bridged between the two contacts. Afterwards, a rGO nanoribbon with the controlled width (typically 20–80 nm) was written between the source and drain electrodes to complete the construction of the device. Theoretical calculations The ensity functional theory calculations were performed using the Vienna Ab initio Simulation Package code [27] , [28] with the exchange correlation functional GGA-PBE [29] . Projector augmented wave potentials were used [30] , and the energy cutoff for the plane-wave basis set was 500 eV. A repeating tetragonal supercell with large lattice constants (26.104 × 17.172 × 26.000 Å 3 ) was adopted. The brillouin zone sampling was carried out using the Monkhorst-Pack grid of (1 × 3 × 1). The supercell contains a Pt 20 cluster surrounded by eight hydrogen atoms and an armchair graphene nanoribbon with an epoxy or a hydroxyl group. The distance between the Pt tip and the underlying GO is about 3 Å. During the optimization, the coordinates of the 16 Pt atoms at the top two layers were fixed, and the heights of the 16 carbon and the 16 hydrogen atoms at the edge of graphene nanoribbon were frozen. The optimization continues until the atom forces were <0.03 eV Å −1 . The climbing image nudged elastic band method [31] was used to explore the adiabatic minimal energy pathway with the minimization of a set of intermediate images. How to cite this article: Zhang, K. et al. Direct writing of electronic devices on graphene oxide by catalytic scanning probe lithography. Nat. Commun. 3:1194 doi: 10.1038/ncomms2200 (2012).